ADAM metalloproteases promote a developmental switch in responsiveness to the axonal repellant Sema3A During embryonic development, axons can gain and lose sensitivity to guidance cues, and this flexibility is essential for the correct wiring of the nervous system. Yet, the underlying molecular mechanisms are largely unknown. Here we show that receptor cleavage by ADAM (A Disintegrin And Metalloprotease) metalloproteases promotes murine sensory axons loss of responsiveness to the chemorepellant Sema3A. Genetic ablation of ADAM10 and ADAM17 disrupts the developmental downregulation of Neuropilin-1 (Nrp1), the receptor for Sema3A, in sensory axons. Moreover, this is correlated with gain of repulsive response to Sema3A. Overexpression of Nrp1 in neurons reverses axonal desensitization to Sema3A, but this is hampered in a mutant Nrp1 with high susceptibility to cleavage. Lastly, we detect guidance errors of proprioceptive axons in ADAM knockouts that are consistent with enhanced response to Sema3A. Our results provide the first evidence for involvement of ADAMs in regulating developmental switch in responsiveness to axonal guidance cues. The basic wiring of the vertebrate nervous system is set up during embryonic development. At this time, newly born neurons project axons over great distances to innervate their targets. Along their pathway axons are directed by guidance cues, either attractive or repulsive [1] . These environmental cues are detected by receptors on specialized cellular sensing structures, termed growth cones, at the growing ends of the axons. Signalling through these receptors modulates growth cone cytoskeletal dynamics and steers the axon’s growth [2] . Axonal growth cones exhibit great developmental plasticity in their response to guidance cues, which is required for their proper guidance. They can lose the ability to respond to a cue that they initially responded to and acquire the ability to react to others [3] , [4] . Often, axons switch responsiveness by modulating the repertoire of receptors expressed at their growth cones [5] , [6] , [7] , [8] , [9] , [10] . Proteolytic release of cell surface proteins, or shedding, has emerged over the past two decades as a key post-translational mechanism for regulating the function of membrane proteins, including receptors [11] , [12] , [13] , [14] . Membrane-anchored metalloproteases (MPs) of the ADAM (A Disintegrin And Metalloprotease) family are major mediators of receptor shedding. Genetic and pharmacological manipulations have demonstrated a requirement for ADAMs for accurate guidance of some axons during development [15] , [16] . Consistent with this, some ADAMs have been shown to cleave axon guidance receptors [17] . As such, they have been implicated in overall control of receptor levels [18] , [19] ; activation of signalling upon ligand binding [20] , [21] ; and disassembly of receptor-ligand complexes [22] , [23] . However, whether metalloproteases regulate the levels of axon guidance receptors as part of a developmental switch in responsiveness is still unknown. The Semaphorin family of guidance cues comprises 27 members across eight subclasses, of which the most studied is the class 3 family of secreted Semaphorins [24] . The receptor complex for the axonal repellant Semaphorin3A (Sema3A) comprises two core elements: Neuropilin-1 (Nrp1), which binds the ligand but lacks signalling capabilities [25] , [26] , [27] , and type-A Plexin, which transmits the signal [28] , [29] . Two other components implicated in activation of the response to Sema3A and endocytosis of the receptor complex, respectively, are the L1 cell adhesion molecule (L1-CAM) and the transiently expressed axonal glycoprotein-1 (TAG-1) [30] , [31] , [32] , [33] . Proprioceptive and cutaneous spinal sensory neurons reside in the dorsal root ganglia (DRG), adjacent to the spinal cord. They project axons that connect target organs of the periphery with the central nervous system. Proprioceptive neurons convey sensory information about muscle contraction and limb position, while cutaneous neurons mediate noxious and innocuous stimuli [34] , [35] . Early during development, Sema3A repels both types of axons. However, as development progresses, proprioceptive axons become insensitive to Sema3A while cutaneous axons remain sensitive [36] , [37] , [38] . This change in responsiveness is correlated with the distinct laminar termination of the two types of fibres. While cutaneous axons terminate in the dorsal spinal cord, proprioceptive axons penetrate into the ventral spinal cord where Sema3A is highly abundant [34] , [36] , [37] , [38] , [39] , [40] . Here we implicate two members of the ADAM family in promoting the developmental loss of responsiveness to Sema3A via cleavage of Nrp1. Genetic ablation of the two ADAMs in the nervous system increases the levels of Nrp1 at growth cones of proprioceptive axons, at a defined developmental stage. This increase is correlated with gain of a repulsive response to Sema3A by these axons. Overexpression of Nrp1 in proprioceptive neurons re-induces responsiveness to Sema3A. This is largely diminished in an Nrp1 mutant with higher susceptibility to cleavage. Finally, the entry of proprioceptive axons into the spinal cord is delayed in ADAM knockouts, in agreement with the delay in loss of responsiveness to Sema3A in vitro . Together, our results establish a role for ADAMs as developmental promoters of switch in axonal responsiveness to guidance cues. Rat proprioceptive axons lose sensitivity to Sema3A at E14 Proprioceptive axons’ loss of responsiveness to Sema3A is a conserved developmental process, which has been demonstrated for mouse and chick [37] , [41] . In rat, proprioceptive axons are already insensitive to Sema3A at embryonic day 14 (E14) [36] . However, it is unclear whether loss of sensitivity occurs at that specific developmental day or even earlier. To resolve this issue, we used the collagen repulsion assay to examine the sensitivity of sensory axons to Sema3A at different embryonic days. In this assay, neuronal explants are embedded in a collagen droplet, next to a cell culture aggregate that secretes the desired repellant. Neurotrophins are added to facilitate growth of the desired axonal subtype. For example, Neurotrophin3 (NT3) and nerve growth factor (NGF) facilitate growth of proprioceptive and cutaneous axons, respectively. Responsiveness to the repellant is evaluated by the axonal growth pattern: radial growth indicates non-responsiveness, while greater axonal growth from the explant side that is distal to the aggregate indicates repulsion. The level of repulsion is represented by a proximal/distal (P/D) ratio, which compares axonal growth on both sides of the explant (low P/D ratio indicates strong repulsion). As can be seen in Fig. 1 , E13 proprioceptive axons grow primarily from the distal side of the DRG explant, indicating strong sensitivity to Sema3A, while E14 and E15 proprioceptive axons grow in a radial manner. In contrast, cutaneous axons exhibit sensitivity to Sema3A at all three stages of development. Thus, we conclude that in the rat, proprioceptive axons switch their responsiveness to Sema3A between E13 and E14. Note that the P/D ratio measured for axons growing in the presence of non-transfected aggregates was slightly higher than 1. This suggests that some minor attractive forces, of unknown nature, may exist between the COS cells and the growing axons. This also underscores the prominence of the repulsive forces exerted on axons by the Sema3A- secreting aggregates, which easily overcome this basal attraction. 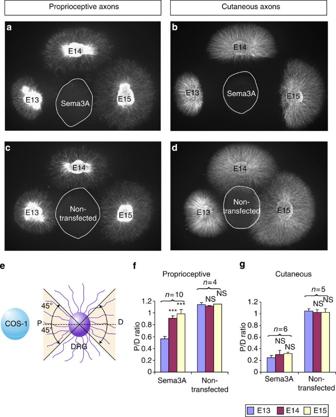Figure 1: Rat proprioceptive axons lose responsiveness to Sema3A at embryonic day 14. DRGs from E13, E14 and E15 rat embryos were embedded in collagen matrix, next to an aggregate of COS-1 cells, either secreting (a,b), or not secreting (c,d), Sema3A. Explants were cultured in the presence of NT3 (a,c), or NGF (b,d), to promote growth of proprioceptive or cutaneous axons, respectively. (e) Scheme illustrating the quantification principals of the assay. For each DRG, axonal length was computationally measured in the range of ±45° around the horizontal axis on both sides of the explant. Total axon length on the DRG side that is proximal (P) to the aggregate was divided by the total axon length on its distal (d) side to obtain a P/D ratio for each explant. Average P/D ratios calculated for proprioceptive and cutaneous axons at the different developmental stages are presented in (f,g), respectively. Results were collected from at least three separate experiments for each condition.n=number of ganglia measured for each developmental stage. Bars represent mean±s.e.m. Mann–WhitneyU-test. ***P<0.001, NS, non significant. DRG, dorsal root ganglion. Figure 1: Rat proprioceptive axons lose responsiveness to Sema3A at embryonic day 14. DRGs from E13, E14 and E15 rat embryos were embedded in collagen matrix, next to an aggregate of COS-1 cells, either secreting ( a , b ), or not secreting ( c , d ), Sema3A. Explants were cultured in the presence of NT3 ( a , c ), or NGF ( b , d ), to promote growth of proprioceptive or cutaneous axons, respectively. ( e ) Scheme illustrating the quantification principals of the assay. For each DRG, axonal length was computationally measured in the range of ±45° around the horizontal axis on both sides of the explant. Total axon length on the DRG side that is proximal (P) to the aggregate was divided by the total axon length on its distal (d) side to obtain a P/D ratio for each explant. Average P/D ratios calculated for proprioceptive and cutaneous axons at the different developmental stages are presented in ( f , g ), respectively. Results were collected from at least three separate experiments for each condition. n =number of ganglia measured for each developmental stage. Bars represent mean±s.e.m. Mann–Whitney U -test. *** P <0.001, NS, non significant. DRG, dorsal root ganglion. Full size image Nrp1 is shed by MPs during the switch in responsiveness In chick, loss of responsiveness to Sema3A correlates with a sharp decrease in Nrp1 levels [41] . To test the relevance of these observations to mammals, we examined Nrp1’s expression in rat embryonic DRG neurons. We used immunofluorescence staining because it enabled us to focus exclusively on growth cones—the cellular compartment where guidance receptors are operating. Thus, our analysis excluded Nrp1 molecules that are highly abundant on the surface of axons [42] , but do not mediate Sema3A signalling [43] . Nrp1 molecules, expressed by Schwann cells and DRG-associated fibroblasts in the culture [44] , were avoided as well. To ensure highly reliable results, immunofluorescence of a large number of growth cones (~1,200–4,500) was measured for each condition. Results of the comparative immunostaining are summarized in Fig. 2 . Overall, we detected a sharp decrease in Nrp1 growth cone levels during the switch in responsiveness. For proprioceptive axonal growth cones, a 43% reduction in Nrp1 immuno-reactivity was observed at E14 (the day of the switch) relative to E13 ( Fig. 2a–c ). These results closely resemble the ~48% reduction that was reported for the chick [41] . Importantly, only a mild decrease was observed for cutaneous axons at E14 and E15 (7 and 5%, respectively), consistent with the continual Sema3A sensitivity of this axonal subtype ( Fig. 2b–c and Supplementary Figure 1a ). 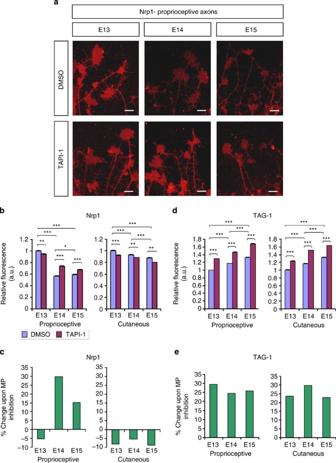Figure 2: Nrp1 is developmentally reduced from the growth cones of proprioceptive axons in a metalloprotease-dependent manner. DRGs were dissected from E13, E14 and E15 rat embryos, and cultured in the presence of the MP inhibitor TAPI-1 (20 μM), or DMSO (carrier). Either NT3 or NGF was added to the cultures to facilitate growth of proprioceptive (aandSupplementary Fig. 1), or cutaneous axons (Supplementary Fig. 1), respectively. After fixation, cultures were surface stained (without permeabilization) against Nrp1 (red) or TAG-1 (green inSupplementary Fig. 1). Relative fluorescence of proprioceptive and cutaneous axonal growth cones at the different developmental stages was measured for both Nrp1 (b) and TAG-1 (d) staining. Mean fluorescence values±s.e.m. for cultures supplemented with TAPI-1 or DMSO are presented in red and blue, respectively. All results were normalized relative to the E13/DMSO value, which was set to 1. For each developmental stage, the percent change in growth cone fluorescence of TAPI-1-supplemented cultures relative to DMSO-supplemented cultures is shown in green (c,e);n(number of growth cones quantified) >1,200 for all conditions. Results for each condition were collected from 3–4 separate experiments. Mann–WhitneyU-test. *P<0.05, **P<0.01, ***P<0.001. Scale bars, 25 μm. MP, metalloproteases; a.u., arbitrary units. Figure 2: Nrp1 is developmentally reduced from the growth cones of proprioceptive axons in a metalloprotease-dependent manner. DRGs were dissected from E13, E14 and E15 rat embryos, and cultured in the presence of the MP inhibitor TAPI-1 (20 μM), or DMSO (carrier). Either NT3 or NGF was added to the cultures to facilitate growth of proprioceptive ( a and Supplementary Fig. 1 ), or cutaneous axons ( Supplementary Fig. 1 ), respectively. After fixation, cultures were surface stained (without permeabilization) against Nrp1 (red) or TAG-1 (green in Supplementary Fig. 1 ). Relative fluorescence of proprioceptive and cutaneous axonal growth cones at the different developmental stages was measured for both Nrp1 ( b ) and TAG-1 ( d ) staining. Mean fluorescence values±s.e.m. for cultures supplemented with TAPI-1 or DMSO are presented in red and blue, respectively. All results were normalized relative to the E13/DMSO value, which was set to 1. For each developmental stage, the percent change in growth cone fluorescence of TAPI-1-supplemented cultures relative to DMSO-supplemented cultures is shown in green ( c , e ); n (number of growth cones quantified) >1,200 for all conditions. Results for each condition were collected from 3–4 separate experiments. Mann–Whitney U -test. * P <0.05, ** P <0.01, *** P <0.001. Scale bars, 25 μm. MP, metalloproteases; a.u., arbitrary units. Full size image In view of previous reports that Nrp1 undergoes ectodomain cleavage by MPs in cell lines [45] , [46] we hypothesized that MPs may also regulate Nrp1 levels in growth cones during embryonic development. Thus, we repeated the Nrp1 staining analyses with rat proprioceptive and cutaneous axons that were cultured in the presence of the broad-spectrum MP inhibitor, TAPI-1 [46] , [47] , [48] , [49] ( Fig. 2 and Supplementary Fig. 1 ). Importantly, a 30% increase in Nrp1 immuno-reactivity was observed in growth cones of proprioceptive axons at E14 upon MP inhibition ( Fig. 2a–c ). At E15 the increase was considerably smaller (~15%), suggesting that Nrp1 shedding peaks at the day of the switch. Notably, no increase in Nrp1 levels was detected upon MP inhibition at E13. Instead, a very modest (5%), but statistically significant, decrease in receptor levels was observed. In cutaneous axonal growth cones, a small decrease in Nrp1 levels was also observed upon MP inhibition, but at all three stages of development ( Fig. 2b,c and Supplementary Fig. 1a ). The cause for this small decrease in both subtypes is unclear, but as TAPI-1 is a broad inhibitor of MPs this may reflect inhibition/activation of biological processes other than ADAM-mediated cleavage. As a negative control, we also measured the relative growth cone levels of TAG-1 ( Fig. 2d,e and Supplementary Fig. 1b,c ). TAG-1 is a cell adhesion molecule that is highly expressed in sensory growth cones and is essential for Sema3A signalling [32] . Our analysis of E13, E14 and E15 sensory growth cones indicated a gradual increase in TAG-1 immunofluorescence in both proprioceptive and cutaneous subtypes ( Fig. 2d ). In addition, TAPI-1 induced a relatively constant increase (~23–30%) in TAG-1 immunoreactivity at all three developmental stages for both proprioceptive and cutaneous axonal growth cones ( Fig. 2e ). Thus, it appears that unlike Nrp1, TAG-1 is constitutively shed by MPs during development. Overall, these results demonstrate close correlation between the dynamic changes in levels of Nrp1 and the sensitivity to Sema3A. They also suggest that MPs contribute to the developmental loss of surface expression of Nrp1 in proprioceptive axonal growth cones. Total Nrp1 is down-regulated in proprioceptive axons Next, we examined whether the decrease in Nrp1 levels at the growth cone during the switch in responsiveness is paralleled by a similar process in the entire axon. We analysed the total levels of Nrp1 in sensory axons by culturing whole DRGs on porous membrane inserts in the presence of NT3 or NGF. In this system, only axons pass through the pores to the bottom part of the membrane. Cell bodies, both neurons and glia, remain restricted to the insert’s upper surface [50] , [51] . Subsequently, each side of the membrane is lysed separately and subjected to western blot analysis. When we compared cell body extracts from NT3-supplemented cultures of E13, E14 and E15 rat DRGs, no significant difference in Nrp1 levels was detected ( Fig. 3a ). However, analysis of axonal extracts, obtained from the same cultures, revealed a substantial decrease in receptor levels, both at E14 and E15 ( Fig. 3b ). Importantly, this decrease was not observed in cutaneous axons, where receptor levels remained constant over the entire time ( Fig. 3c ). Finally, we tested whether Nrp1’s downregulation in E14 and E15 proprioceptive axons is mediated by MPs. However, no significant increase in the total receptor levels was observed upon addition of TAPI-1 to these cultures ( Fig. 3d ). Together, these results suggest the existence of a gradual process for downregulation of total Nrp1 levels in proprioceptive axons. Interestingly, the decrease in total receptor levels proceeds even at E15, 1 day after the switch in responsiveness to Sema3A. Our results provide no evidence for the involvement of MPs in this process. However, this may result from the limited resolution of the biochemical analysis, which reflects total axonal contents, rather than axonal membrane composition. Overall, these results suggest that an additional global MP-independent mechanism(s) accompanies the shedding of Nrp1 at the growth cone. 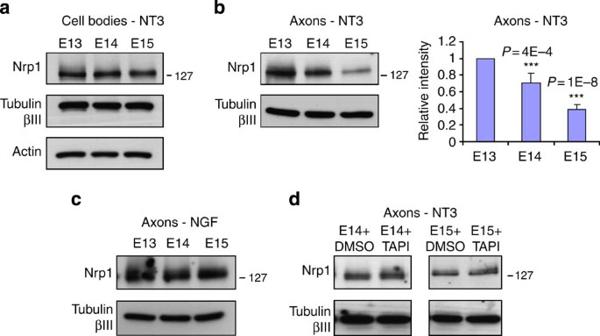Figure 3: Nrp1 is developmentally downregulated in proprioceptive axons. E13, E14 and E15 DRGs were grown on cell culture inserts. NT3 (a,b,d) or NGF- (c) were added to the culture media to promote growth of proprioceptive or cutaneous axons, respectively. Cell bodies (a) and axons (b–d) were extracted separately from the two sides of the insert membrane and analysed by western blot with antibodies against Nrp1. (d) E14 and E15 cultures were supplemented with the MP inhibitor TAPI-1 or DMSO (carrier). Immunoblots for tubulin βIII (neuronal specific) and actin were used as loading controls. Molecular weight markers (kDa) are indicated on the right. Full-scanned western blots are presented inSupplementary Fig. 6. The quantification of western blot results inbis based on five separate experiments. Bars represent mean±s.d. Two-tailed Student’st-test. ***P<0.001. Figure 3: Nrp1 is developmentally downregulated in proprioceptive axons. E13, E14 and E15 DRGs were grown on cell culture inserts. NT3 ( a , b , d ) or NGF- ( c ) were added to the culture media to promote growth of proprioceptive or cutaneous axons, respectively. Cell bodies ( a ) and axons ( b – d ) were extracted separately from the two sides of the insert membrane and analysed by western blot with antibodies against Nrp1. ( d ) E14 and E15 cultures were supplemented with the MP inhibitor TAPI-1 or DMSO (carrier). Immunoblots for tubulin βIII (neuronal specific) and actin were used as loading controls. Molecular weight markers (kDa) are indicated on the right. Full-scanned western blots are presented in Supplementary Fig. 6 . The quantification of western blot results in b is based on five separate experiments. Bars represent mean±s.d. Two-tailed Student’s t -test. *** P <0.001. Full size image Nrp1 is a substrate for both ADAM10 and ADAM17 Members of the ADAM family are major regulators of receptor shedding [13] , [14] . Furthermore, ADAM10 has been shown to cleave Nrp1 in transfected COS-7 cells and in mouse embryonic fibroblasts [45] . Thus, to identify candidate MPs that may catalyse Nrp1’s shedding at the growth cone, we decided to focus on ADAMs and test their ability to cleave the receptor in cell culture. First, we ectopically expressed Nrp1, Flag-tagged on its N-terminal (extracellular) end, in HEK293T cells. In a western blot analysis of the culture’s supernatant with antibodies against the Flag epitope a single band, corresponding to the extracellular fragment of Nrp1, was detected ( Fig. 4a ). This band largely disappeared when the cells were incubated with TAPI-1 (88% decrease). Cleavage was also blocked by the pharmacological agent GI254023X (89% reduction), which inhibits ADAM10 (but also matrix metalloproteases) [52] . Finally, Nrp1’s shedding was considerably reduced when it was co-transfected with shRNA construct directed against ADAM10, but not with a control shRNA ( Fig. 4b ). Together, these results indicate that endogenous ADAM10 mediates the constitutive cleavage of Nrp1 in this cell line. 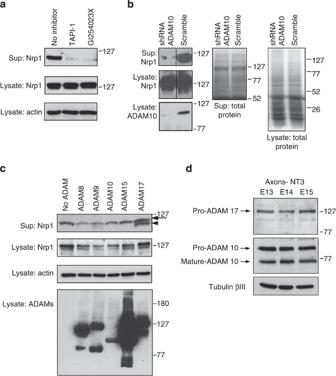Figure 4: Nrp1 is cleaved by ADAM10 and ADAM17. (a) HEK-293T cells were transfected with plasmids encoding Nrp1, Flag-tagged on its extracellular (N-terminal) end. Cultures were supplemented with TAPI-1 (20 μM), GI254023X (5 μM) or DMSO (carrier). After 24 h incubation, supernatants (sup) were analysed by western blot with antibodies against the Flag epitope for the presence of Nrp1’s ectodomain. (b) Flag-Nrp1 and shRNA constructs targeting ADAM10, or scramble shRNA as control, were co-transfected into HEK293T cells. Nrp1 levels both in the supernatants and lysates were analysed by western blot against the Flag epitope. shRNA silencing efficiency was validated by examining the lysates for ADAM10 expression levels. Total protein coomassie staining of both the sup and the lysate served as loading control. (c) Flag-tagged Nrp1 and five Myc-tagged ADAMs, or an empty vector as control, were co-transfected into HEK293T cells. Supernatants and cell lysates were analysed by western blot with antibodies against the Flag epitope, the Myc epitope and actin, as indicated. The constitutive (ADAM10) cleavage product is indicated by an arrow. ADAM17 cleavage product is marked by an arrowhead. In the anti-Myc (ADAMs) immunoblot, where two bands appear in a single lane, the upper band represents the ADAM pro-protein, while the lower indicates the mature and active MP. (d) Extracts of E13, E14 and E15 proprioceptive axons obtained from DRG insert cultures were analysed by western blot with antibodies against ADAM10 (middle) and ADAM17 (up). Anti-tubulin βIII (neuronal specific) immunoblot (down) served as a loading control. Molecular weight markers (kDa) are indicated on the right. Full-scanned western blots are presented inSupplementary Fig. 7. Figure 4: Nrp1 is cleaved by ADAM10 and ADAM17. ( a ) HEK-293T cells were transfected with plasmids encoding Nrp1, Flag-tagged on its extracellular (N-terminal) end. Cultures were supplemented with TAPI-1 (20 μM), GI254023X (5 μM) or DMSO (carrier). After 24 h incubation, supernatants (sup) were analysed by western blot with antibodies against the Flag epitope for the presence of Nrp1’s ectodomain. ( b ) Flag-Nrp1 and shRNA constructs targeting ADAM10, or scramble shRNA as control, were co-transfected into HEK293T cells. Nrp1 levels both in the supernatants and lysates were analysed by western blot against the Flag epitope. shRNA silencing efficiency was validated by examining the lysates for ADAM10 expression levels. Total protein coomassie staining of both the sup and the lysate served as loading control. ( c ) Flag-tagged Nrp1 and five Myc-tagged ADAMs, or an empty vector as control, were co-transfected into HEK293T cells. Supernatants and cell lysates were analysed by western blot with antibodies against the Flag epitope, the Myc epitope and actin, as indicated. The constitutive (ADAM10) cleavage product is indicated by an arrow. ADAM17 cleavage product is marked by an arrowhead. In the anti-Myc (ADAMs) immunoblot, where two bands appear in a single lane, the upper band represents the ADAM pro-protein, while the lower indicates the mature and active MP. ( d ) Extracts of E13, E14 and E15 proprioceptive axons obtained from DRG insert cultures were analysed by western blot with antibodies against ADAM10 (middle) and ADAM17 (up). Anti-tubulin βIII (neuronal specific) immunoblot (down) served as a loading control. Molecular weight markers (kDa) are indicated on the right. Full-scanned western blots are presented in Supplementary Fig. 7 . Full size image Next, we co-expressed Nrp1 with several members of the ADAM family that were previously implicated in receptor shedding and analysed the supernatants ( Fig. 4c ). For all ADAMs, except ADAM17, a single band, corresponding to Nrp1’s cleaved form, was observed. The band was similar in migration and comparable in intensity to the band observed when Nrp1 was co-expressed with an empty vector. Therefore, at least in this system, those overexpressed ADAMs do not enhance the constitutive (endogenous ADAM10-mediated) Nrp1 shedding. The co-expression with ADAM10 did not increase shedding levels, presumably due to the low efficiency of ADAM10 overexpression (see total ADAM expression, Fig. 4c ). In contrast, co-expression with ADAM17 yielded an additional band, which migrated faster than the ADAM10 cleavage product. This result suggests that ADAM17 can also cleave Nrp1, but apparently at a site that is more distant from the cell membrane than the one used by ADAM10. To ensure that both candidate ADAMs are actually expressed in axons, we examined their presence in extracts of rat E13, E14 and E15 proprioceptive axons, obtained from DRG insert cultures ( Fig. 4d ). Western blot analysis with antibodies against ADAM10 and ADAM17 confirmed the presence of both ADAMs in axons. ADAM10 was identified both in its pro-protein and mature/active forms. ADAM17 was observed primarily in its pro-form. The expression levels of ADAMs appeared constant throughout the entire developmental period. Higher Nrp1 levels and Sema3A sensitivity in ADAM KO axons Next, we examined the contribution of ADAM10 and ADAM17 to the loss of sensitivity to Sema3A by genetic inactivation of the two genes in the mouse nervous system. In mice, the developmental stage that parallels rat E14 (and the loss of sensitivity to Sema3A) is reached at E12.5. Previously, it has been reported that mouse proprioceptive axons lose responsiveness to Sema3A at E14.5 (ref. 37 ). However, collagen assays we performed indicated that this process takes place already at E12.5 ( Supplementary Fig. 2 ). First, we wanted to test the effect of the two ADAMs’ elimination on Nrp1’s expression levels at the growth cones of proprioceptive axons. For this purpose, ADAM10, ADAM17 and ADAM10/17 conditional knockout (cKO) embryos were generated (Cre recombinase was under control of the Nestin promoter). DRGs from wild type and mutant embryos were cultured in the presence of NT3 and immunostained with antibodies against Nrp1 ( Fig. 5 ). Nrp1 immunoreactivity of wild-type axonal growth cones was 27% lower at E12.5 than at E11.5 ( Fig. 5a,d,i ). This expected decrease correlates with the loss of sensitivity to Sema3A, although it is more moderate than the one observed in chick and rat. When MP activity was inhibited by TAPI-1 at E12.5, a substantial 35% increase in Nrp1 levels was observed ( Fig. 5e,i,j ). Importantly, at E11.5 no significant increase in receptor levels was detected on MP inhibition ( Fig. 5b,i,j ), highlighting the specificity of Nrp1’s cleavage to the day of the switch. For each of the single knockouts, only a small increase in Nrp1 levels was detected at E12. (5% for ADAM17 cKO and 7% for ADAM10 cKO) ( Fig. 5f,g,i,j ). However, Nrp1 levels in growth cones of the ADAM10/17 double-knockout axons increased by 25% at E12.5, mimicking most of the effect achieved by the pharmacological agent ( Fig. 5h–j ). Notably, at E11.5 only a small increase (6%) was detected in Nrp1 levels in double-knockout growth cones, relative to wild-type counterparts. Overall, these findings suggest that ADAM10 and 17 are the two major MPs that catalyse Nrp1 shedding at growth cones of proprioceptive axons during the switch in responsiveness to Sema3A. 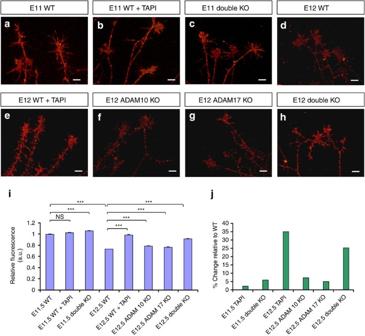Figure 5: ADAM10/17 double-knockout proprioceptive axons exhibit increased levels of Nrp1 at their growth cones. DRGs were dissected from E11.5 (a–c) and E12.5 (d–h) mice embryos of four different genotypes—wild type, ADAM10 cKO, ADAM17 cKO and ADAM10/17 double cKO. Explants were cultured in the presence of NT3 to facilitate growth of proprioceptive axons. Wild-type DRGs were cultured either with (b,e) or without (a,d) TAPI-1 (20 μM). Cultures of all four genotypes without TAPI-1 were supplemented with equivalent volumes of DMSO (carrier). Following fixation, the samples were surface stained (without permeabilization) with antibodies against Nrp1. (i) Relative fluorescence of growth cones from the different genotypes was measured. Results were normalized relative to average fluorescence of E11.5 wild-type growth cones with DMSO, which was set to 1;n(number of growth cones quantified) >1,200 for each condition. Results for each condition were collected from 3 to 7 separate experiments. (j) Growth cone fluorescence of mutant or pharmacologically inhibited neurons was compared with that of wild-type growth cones of the same embryonic day. Bars represent mean±s.e.m. Mann–WhitneyU-test. ***P<0.001, NS, non significant. Scale bars, 25 μm. cKO, conditional knockout. Figure 5: ADAM10/17 double-knockout proprioceptive axons exhibit increased levels of Nrp1 at their growth cones. DRGs were dissected from E11.5 ( a – c ) and E12.5 ( d – h ) mice embryos of four different genotypes—wild type, ADAM10 cKO, ADAM17 cKO and ADAM10/17 double cKO. Explants were cultured in the presence of NT3 to facilitate growth of proprioceptive axons. Wild-type DRGs were cultured either with ( b , e ) or without ( a , d ) TAPI-1 (20 μM). Cultures of all four genotypes without TAPI-1 were supplemented with equivalent volumes of DMSO (carrier). Following fixation, the samples were surface stained (without permeabilization) with antibodies against Nrp1. ( i ) Relative fluorescence of growth cones from the different genotypes was measured. Results were normalized relative to average fluorescence of E11.5 wild-type growth cones with DMSO, which was set to 1; n (number of growth cones quantified) >1,200 for each condition. Results for each condition were collected from 3 to 7 separate experiments. ( j ) Growth cone fluorescence of mutant or pharmacologically inhibited neurons was compared with that of wild-type growth cones of the same embryonic day. Bars represent mean±s.e.m. Mann–Whitney U -test. *** P <0.001, NS, non significant. Scale bars, 25 μm. cKO, conditional knockout. Full size image Next, we used the collagen repulsion assay to test whether the increase in Nrp1 levels in the ADAM knockouts has functional consequences. As can be seen in Fig. 6a–c,f a mild increase in sensitivity to Sema3A was observed for both ADAM10 and ADAM17 single cKOs (17% and 15% decrease in P/D ratio, respectively) at E12.5. However, when ADAM10/17 double-cKO DRGs were tested in the same experimental system, a considerable increase in sensitivity was observed (33% decrease in P/D ratio). Interestingly, the difference in sensitivity between wild-type and double-knockout axons was not observed at E13.5 ( Fig. 6d,f ), implying that a parallel molecular process, independent of ADAM10 and 17, ensures axonal desensitization with a 1 day delay—likely the decrease in total Nrp1 described above. Overall, these results demonstrate that combined ablation of ADAM10 and 17 re-sensitizes proprioceptive axons to Sema3A, consistent with the increased levels of Nrp1 at their growth cones. 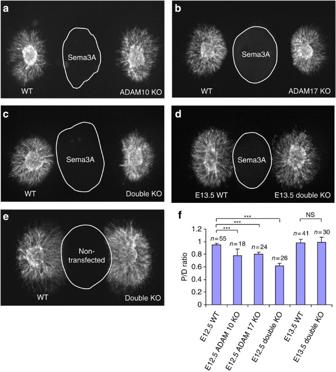Figure 6: ADAM10/17 double-knockout proprioceptive axons exhibit increased sensitivity to Sema3As. Wild type and mutant proprioceptive neurons were tested in collagen repulsion assay for sensitivity to Sema3A. DRGs were dissected from wild type, ADAM10 cKO (a), ADAM17 cKO (b) and ADAM10/17 double cKO (c,e) mice embryos at E12.5, or wild type and ADAM10/17 double cKO embryos at E13.5 (d). Explants were embedded in collagen matrix, next to Sema3A-secreting- (a–d) or non-transfected (e) aggregates of COS-1 cells, as indicated. Each droplet of collagen harbored a pair of wild type and mutant DRGs, originating from littermate embryos. Culture media were supplemented with NT3 to support the growth of proprioceptive axons. (f) P/D ratio quantification for wild type and mutant DRGs, cultured in the presence of Sema3A-secreting aggregates. Results were collected from 3 to 6 separate experiments for each condition;n=number of ganglia measured for each condition. Bars represent mean±s.e.m. Mann–WhitneyU-test. ***P<0.001; NS, non significant. Figure 6: ADAM10/17 double-knockout proprioceptive axons exhibit increased sensitivity to Sema3As. Wild type and mutant proprioceptive neurons were tested in collagen repulsion assay for sensitivity to Sema3A. DRGs were dissected from wild type, ADAM10 cKO ( a ), ADAM17 cKO ( b ) and ADAM10/17 double cKO ( c , e ) mice embryos at E12.5, or wild type and ADAM10/17 double cKO embryos at E13.5 ( d ). Explants were embedded in collagen matrix, next to Sema3A-secreting- ( a – d ) or non-transfected ( e ) aggregates of COS-1 cells, as indicated. Each droplet of collagen harbored a pair of wild type and mutant DRGs, originating from littermate embryos. Culture media were supplemented with NT3 to support the growth of proprioceptive axons. ( f ) P/D ratio quantification for wild type and mutant DRGs, cultured in the presence of Sema3A-secreting aggregates. Results were collected from 3 to 6 separate experiments for each condition; n =number of ganglia measured for each condition. Bars represent mean±s.e.m. Mann–Whitney U -test. *** P <0.001; NS, non significant. Full size image Overexpression of Nrp1 induces sensitivity to Sema3A To further establish that downregulation of Nrp1 is the cause for the loss of responsiveness to Sema3A, we overexpressed the receptor in non-responsive rat proprioceptive neurons and tested the effect on axonal sensitivity. To obtain high yields of transfection, E14 DRGs were dissociated into single cells, electroporated with plasmids encoding Flag-tagged Nrp1 and concentrated again to form neuronal aggregates ( Fig. 7a ). These aggregates were tested in collagen assays, parallel to neuronal aggregates overexpressing Flag-tagged L1-CAM. This adhesion molecule was selected as a control because it is another essential component of the receptor complex for Sema3A, and it is a known substrate of both ADAM10 and 17 (refs 53 , 54 ). 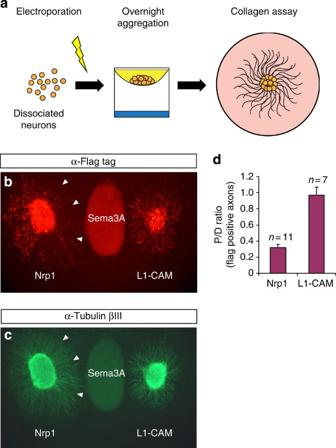Figure 7: Overexpression of Nrp1 sensitizes proprioceptive axons to Sema3A. (a) General scheme illustrating the generation of neuronal aggregates. DRGs are dissociated, electroporated with plasmids encoding the desired receptor, and incubated overnight in a ‘hanging drop’. The newly formed neuronal aggregates are tested the following day in collagen assay. (b,c) Neuronal aggregates, overexpressing either Nrp1 or L1-CAM, Flag tagged at their (extracellular) N-termini, were prepared from E14 rat DRGs. The two types of aggregates were embedded in collagen next to Sema3A-secreting aggregate of COS-1 cells, as indicated. NT3 was added to the cultures to facilitate growth of proprioceptive axons. After incubation, cultures were fixed and stained for tubulin βIII (c, green) to visualize all the axons. The subpopulations of axons overexpressing Nrp1 (left aggregate) or L1-CAM (right aggregate) were visualized using anti-Flag staining (b, red). Arrowheads indicate representative proximal axons (positive for tubulin βIII) that are clearly negative for Flag-tagged Nrp1. (d) P/D ratios calculated for axons overexpressing Nrp1 or L1-CAM (Flag positive axons).n=number of neuronal aggregates measured. Bars represent mean±s.e.m. Figure 7: Overexpression of Nrp1 sensitizes proprioceptive axons to Sema3A. ( a ) General scheme illustrating the generation of neuronal aggregates. DRGs are dissociated, electroporated with plasmids encoding the desired receptor, and incubated overnight in a ‘hanging drop’. The newly formed neuronal aggregates are tested the following day in collagen assay. ( b , c ) Neuronal aggregates, overexpressing either Nrp1 or L1-CAM, Flag tagged at their (extracellular) N-termini, were prepared from E14 rat DRGs. The two types of aggregates were embedded in collagen next to Sema3A-secreting aggregate of COS-1 cells, as indicated. NT3 was added to the cultures to facilitate growth of proprioceptive axons. After incubation, cultures were fixed and stained for tubulin βIII ( c , green) to visualize all the axons. The subpopulations of axons overexpressing Nrp1 (left aggregate) or L1-CAM (right aggregate) were visualized using anti-Flag staining ( b , red). Arrowheads indicate representative proximal axons (positive for tubulin βIII) that are clearly negative for Flag-tagged Nrp1. ( d ) P/D ratios calculated for axons overexpressing Nrp1 or L1-CAM (Flag positive axons). n =number of neuronal aggregates measured. Bars represent mean±s.e.m. Full size image Collagen cultures were stained for both the Flag tag and the axonal marker tubulin-βIII. Since not all the cells undergo transfection, only a subset of tubulin-βIII-positive axons is also positive for the Flag tag. For both types of neuronal aggregates, overall axonal growth was radial ( Fig. 7c ), as expected for rat proprioceptive neurons at E14. Radial growth was also observed in the subpopulation of axons overexpressing L1-CAM ( Fig. 7b right). In contrast, axons overexpressing Nrp1 projected very few axons in the direction of the Sema3A-secreting cells ( Fig. 7b left), indicating they are highly sensitive to the repellant These results strongly support the identification of Nrp1 as the receptor component whose cleavage causes the loss of sensitivity to Sema3A. Hampered sensitizing ability in Nrp1 hyper-cleavable mutant To obtain further support for the ADAM-mediated cleavage mechanism, we attempted to generate mutant Nrp1s with altered shedding features. Occasionally, short modifications in the juxtamembrane region of ADAM substrates, close to the cleavage site, have a marked effect on their shedding efficiency [22] . Since no consensus cleavage sequence for ADAMs has been identified to date [13] , [14] , our first step was to crudely map the ADAM10 and ADAM17 cleavage sites in Nrp1. This was achieved by insertion of the Myc epitope at different locations along the receptor’s juxtamembrane region and analysis of the cleavage products by western blot (for details—see Supplementary Methods section). Using this approach, we mapped the ADAM10 cleavage site close to residue 840 of Nrp1. The ADAM17 cleavage site was positioned N-terminally to residue 824 ( Supplementary Fig. 10 ). Next, we generated a set of Nrp1 mutants with short deletions near the identified cleavage sites. Each mutant was expressed in HEK293T cells, and the amount ADAM10 or ADAM17-mediated cleavage product was compared with that of the wild-type receptor. Overall, two mutants with ‘hyper-cleavable’ (h.c.) phenotype were identified. Nrp1-lacking residues 786–790, designated ADAM17 h.c., exhibited a fivefold increase in ADAM17 (but not ADAM10) cleavage relative to wild type ( Fig. 8a left). In contrast, Nrp1-lacking residues 835-839, designated ADAM10 h.c., was fivefold more susceptible to ADAM10 (but not ADAM17) cleavage ( Fig. 8a right). Overall expression of both mutants and their ability to reach the cell membrane were not affected by the deletions (lysates in Fig. 8a and Supplementary Fig. 3a ). Furthermore, their ability to bind Sema3A, interact with Plexin-A1 or Plexin-A4 (the Nrp1 signalling co-receptors), or to dimerize with other Nrp1 or Neuropilin-2 (Nrp2) molecules was also not impaired ( Supplementary Fig. 3b–f ). 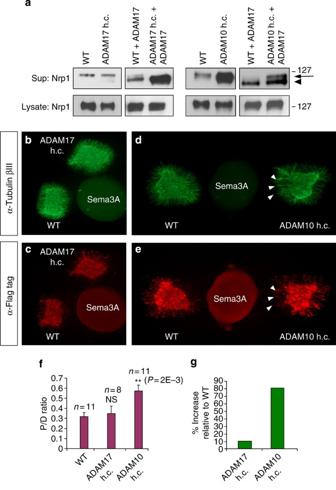Figure 8: Enhanced cleavage of Nrp1 hampers its ability to induce sensitivity to Sema3A. (a) HEK293T cells were transfected with wild-type Nrp1 or the mutant receptors ADAM10 hyper-cleavable (h.c.) and ADAM17 hyper-cleavable. All three constructs harboured Flag tag at their (extracellular) N-termini. Supernatants (sup) were collected and analysed by western blot to evaluate cleavage efficiency by ADAM10. Similar analysis was performed on supernatants of cells, co-transfected with the different Nrp1s and ADAM17. ADAM10 and ADAM17 cleavage products are indicated by arrow and arrowhead, respectively. Full-scanned blots are presented inSupplementary Fig. 8. (b–e) Neuronal aggregates overexpressing wild-type Nrp1, ADAM10 h.c., or ADAM17 h.c. were prepared from rat E14 DRGs and cultured in the presence of NT3. Aggregates were tested in collagen assay for sensitivity to Sema3A. After fixation, cultures were immunostained against tubulin βIII to visualize all axons (b,d, green). Axons overexpressing the different Nrp1 variants were visualized using anti-Flag staining (c,e, red). Arrowheads indicate representative proximal axons that clearly overexpress the ADAM10 h.c. Nrp1. (f) Mean P/D ratios±s.e.m for aggregates overexpressing wild-type and mutant Nrp1s;n=number of neuronal aggregates measured. (g) Percent increase in mean P/D ratios of the hyper-cleavable mutants relative to wild-type Nrp1. Mann–WhitneyU-test. **P<0.01. NS, non significant. Figure 8: Enhanced cleavage of Nrp1 hampers its ability to induce sensitivity to Sema3A. ( a ) HEK293T cells were transfected with wild-type Nrp1 or the mutant receptors ADAM10 hyper-cleavable (h.c.) and ADAM17 hyper-cleavable. All three constructs harboured Flag tag at their (extracellular) N-termini. Supernatants (sup) were collected and analysed by western blot to evaluate cleavage efficiency by ADAM10. Similar analysis was performed on supernatants of cells, co-transfected with the different Nrp1s and ADAM17. ADAM10 and ADAM17 cleavage products are indicated by arrow and arrowhead, respectively. Full-scanned blots are presented in Supplementary Fig. 8 . ( b – e ) Neuronal aggregates overexpressing wild-type Nrp1, ADAM10 h.c., or ADAM17 h.c. were prepared from rat E14 DRGs and cultured in the presence of NT3. Aggregates were tested in collagen assay for sensitivity to Sema3A. After fixation, cultures were immunostained against tubulin βIII to visualize all axons ( b , d , green). Axons overexpressing the different Nrp1 variants were visualized using anti-Flag staining ( c , e , red). Arrowheads indicate representative proximal axons that clearly overexpress the ADAM10 h.c. Nrp1. ( f ) Mean P/D ratios±s.e.m for aggregates overexpressing wild-type and mutant Nrp1s; n =number of neuronal aggregates measured. ( g ) Percent increase in mean P/D ratios of the hyper-cleavable mutants relative to wild-type Nrp1. Mann–Whitney U -test. ** P <0.01. NS, non significant. Full size image Subsequently, we tested the ability of the ‘hyper-cleaveable’ mutants to induce sensitivity to Sema3A. In theory, the sensitizing effect of Nrp1’s overexpression should be compromised in the ‘hyper-cleavable’ mutants, since much of the ectopically expressed receptor is subjected to cleavage. To examine this prediction, neuronal aggregates, overexpressing wild type or mutant Nrp1, were tested in collagen assay. As expected for rat E14 proprioceptive neurons, the gross axonal projection pattern for all three types of aggregates was radial ( Fig. 8b,d ). The subpopulation of neurons overexpressing the ADAM17 h.c. mutant projected axons almost exclusively from the distal side ( Fig. 8c ), very much like neurons overexpressing the wild-type receptor. In contrast, neurons overexpressing ADAM10 h.c. projected axons in a much more radial manner, indicating reduced sensitivity ( Fig. 8e–g ). These results support the role of Nrp1 ectodomain shedding in the loss of responsiveness to Sema3A. They also imply that ADAM10 may play a more dominant role in cleaving Nrp1 in growth cones of proprioceptive axons than ADAM17. ADAM KO axons exhibit delayed entry into the spinal cord As a first step towards determining the physiological significance of the MP-mediated downregulation of Nrp1, we compared the spinal projections of proprioceptive neurons in wild type and ADAM knockout mouse embryos. As mentioned above, Sema3A is secreted from the ventral parts of the spinal cord, restricting the dorso-ventral progress of sensory afferents that remain responsive to it. Accordingly, our model predicts that the advance of proprioceptive axons through the spinal cord will be hindered in the ADAM10/17 double-knockout embryos, due to their increased sensitivity to Sema3A. To examine this issue, transverse cryo-sections of wild type and mutant spinal cords were stained against Trk-C (the receptor for NT3) to visualize the proprioceptive fibres ( Fig. 9 ). At E12.5, when the switch in responsiveness is observed in vitro , proprioceptive axons, in both wild type and double-knockout embryos, can be detected at the dorsal rim of the spinal cord ( Fig. 9a,b,i ). One day later, at E13.5, these axons have already penetrated deep into the cord, progressing ventrally in parallel to the midline ( Fig. 9c,i ). Strikingly, in the ADAM10/17 double-knockout embryos these fibres are entirely excluded from the spinal cord and remain restricted to its dorsal rim ( Fig. 9d,i ), a result that fits our model. Interestingly, by E14.5 the double-knockout afferents no longer avoid the cord, but instead penetrate it robustly ( Fig. 9f,i ). To some extent these fibres appear more diffuse than normal, but the extent of their growth into the cord seems to resemble wild-type counterparts ( Fig. 9e,f,i ). This again fits our in vitro observations, which indicated a 1 day delay in the loss of responsiveness of the double-knockout axons. 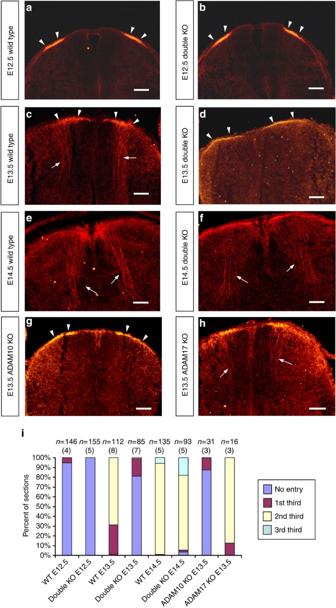Figure 9: Genetic elimination of ADAM10 in the nervous system delays entry of sensory axons into the spinal cord. (a–h) Transverse cervical spinal cord cryosections from wild type, ADAM10 cKO, ADAM17 cKO and ADAM10/17 double-cKO embryos at E12.5, E13.5 and E14.5, as indicated. Sections were immunostained with antibodies against TrkC to visualize proprioceptive axons. Proprioceptive axons accumulating at the spinal cord’s dorsal rim are indicated by arrowheads. Dorso-ventral proprioceptive projections into the spinal cord are indicated by arrows. (i) Spinal cord penetration index. All cryo sections were divided into categories according to the termination site of the longest TrkC+fibre: no entry—blue; 1st third of the spinal cord (dorsal)—red; 2nd third (mid)—pale yellow; 3rd third (ventral)—pale blue. Results for all genotypes/ developmental stages are summarized in a 100% stacked column;n=number of sections used for the quantifications (number in parentheses indicates number of dissected embryos). Bars, 100 μM. Dorsal is up. Figure 9: Genetic elimination of ADAM10 in the nervous system delays entry of sensory axons into the spinal cord. ( a – h ) Transverse cervical spinal cord cryosections from wild type, ADAM10 cKO, ADAM17 cKO and ADAM10/17 double-cKO embryos at E12.5, E13.5 and E14.5, as indicated. Sections were immunostained with antibodies against TrkC to visualize proprioceptive axons. Proprioceptive axons accumulating at the spinal cord’s dorsal rim are indicated by arrowheads. Dorso-ventral proprioceptive projections into the spinal cord are indicated by arrows. ( i ) Spinal cord penetration index. All cryo sections were divided into categories according to the termination site of the longest TrkC + fibre: no entry—blue; 1st third of the spinal cord (dorsal)—red; 2nd third (mid)—pale yellow; 3rd third (ventral)—pale blue. Results for all genotypes/ developmental stages are summarized in a 100% stacked column; n =number of sections used for the quantifications (number in parentheses indicates number of dissected embryos). Bars, 100 μM. Dorsal is up. Full size image We also examined the trajectory of proprioceptive axons in the single-knockout embryos at E13.5. In ADAM17 single knockouts, TrkC-positive axons entered the spinal cord on schedule ( Fig. 9h,i ). In contrast, in ADAM10 knockouts proprioceptive fibres were excluded from the cord just like the double-knockout fibres ( Fig. 9g,i ). In this regard, the in vivo results differ from the in vitro observations, which attributed only a mild increase in Sema3A-sensitivity to both single knockouts. These results could be explained if in vivo other factors influence the degree of responsiveness of the single-knockout axons, and/or the in vitro assay provides an imperfect measure of the precise extent to which the axons acquire responsiveness. Alternatively, we cannot exclude that the phenotypes in the mutants reflect effects that are not autonomous to the proprioceptive neurons. For example, overall morphological inspection of double-knockout spinal cords at E13.5 revealed that their central canal does not form ( Supplementary Fig. 4b ) (possibly due to defective Notch signalling in the Nestin-positive progenitor cells at the midline). In principal, such defects may produce a non-permissive environment for axonal growth, or the lack of axonal attractants, possibly accounting for the observed phenotype. However, this seems less likely to be the case, since mutant axons exhibit no difficulty in entering the cord 1 day later, at E14.5, while the morphological abnormalities persist even at E15.5 ( Supplementary Fig. 4d ). Finally, we examined whether axons that exhibit pathfinding errors in embryos with defective Sema3A signalling (namely the Sema3A, Nrp1 and Plexin-A mutants [25] , [29] , [55] , [56] ) also misproject in ADAM10/17 double-knockout embryos. Contrary to the former mutants, whose axons extend beyond their normal targets due to lack of Sema3A inhibitory signalling, axonal projections of the ADAM knockouts are expected to be more restricted than wild type due to increased sensitivity to the repellant. That said, the misprojections in the Sema3A-related mutants are primarily derived from NGF-dependent neurons. Since we have demonstrated ( Fig.2 and Supplementary Fig. 1 ) that there is no MP-dependent downregulation of Nrp1 in these neurons, our model does not predict pathfinding defects for this subtype of axons in the ADAM knockouts. In agreement, the overall axonal growth and patterns in the ADAM10 −/− /ADAM17 −/− embryo were similar to wild type as observed by whole mount anti-neurofilament staining ( Supplementary Fig. 5 ). Together, these observations highlight the specificity of the guidance phenotype identified for proprioceptive axons entering the spinal cord. During embryonic development, DRG neurons project axons that innervate the spinal cord in a highly stereospecific manner. Two sets of repellents have been implicated in shaping the topographic organization of sensory axons in the spinal cord. Proprioceptive fibres, which exclusively express the PlexinA1 receptor, are restricted from the superficial dorsal horn by the chemorepellants Sema6C and Sema6D [57] . In contrast, cutaneous fibres are confined to the dorsal horn by Sema3A, which is widely expressed throughout the rest of the spinal cord [36] , [37] , [38] . In early stages of development, proprioceptive axons are also repelled by Sema3A. However, as they penetrate the spinal cord and progress towards their ventral targets, these axons lose sensitivity to the repellant by downregulating its receptor, Nrp1 [40] , [41] . Here we show that downregulation of Nrp1 is facilitated by ADAM MPs, which cleave the receptor from the surface of growth cones at a precise developmental time point. Genetic ablation of ADAMs in the nervous system causes a 1 day delay in the loss of responsiveness to Sema3A both in vitro and in vivo . The complete physiological significance of this delay remains unresolved, since Nestin-Cre ADAM10 cKOs die at birth [58] . Thus, full assessment of the delay’s implications on the correct wiring of proprioceptive fibres awaits the generation of more specific conditional knockouts. Previous studies have uncovered important aspects of MP contribution to axon guidance. One major aspect is the catalysis of structural changes that are essential for the proper functioning of guidance receptors [21] , [22] , [23] . Another role, suggested by two previous studies, is the control of axonal sensitivity through regulation of receptor levels. One work reported MP-dependent shedding of DCC, the receptor for Netrin, which mediates attractive signalling in commissural axons [18] . The other demonstrated that ADAM17-mediated cleavage of Neogenin, a receptor for Netrin and the repulsive guidance molecule (RGM), promotes RGM repulsive response in cortical neurons [19] . In both cases, MP inhibition affected overall axonal outgrowth in the presence of the ligand. However, the temporal context in these two studies remained unclear. It was not determined whether the observed MP activity is induced at a certain point during development or instead fulfills some constitutive ‘housekeeping’ role. In our system, the ADAM-mediated shedding is triggered only in a specific type of cells, at a specific developmental stage. Therefore, our data provide the first demonstration that shedding of guidance receptors mediates axonal switch in responsiveness as part of a developmental programme. Developmental events that involve switch in responsiveness to guidance cues have been studied in many systems—most of all in commissural axons and retinal ganglion cells. These studies reveal that axons use diverse strategies to modulate receptor levels at their growth cones, as a means to control sensitivity. Transcriptional control [59] , receptor sorting and trafficking [5] , [7] , intra-cellular proteolysis [9] and endocytosis [8] are only some of the mechanisms described. Here we describe another mechanism—ectodomain shedding by metallproteases—that can contribute to eliminating receptor molecules from the cell surface. Two features distinguish ectodomain shedding from other mechanisms used by axons to downregulate receptors (for example, repression of transcription, endocytosis). First, it involves active elimination of receptor molecules, rather than gradual degradation or ligand-binding-dependent internalization. Moreover, the soluble ectodomain produced as a cleavage byproduct may serve as a decoy to sequester ligand (see for example ref. 60 ). Second, it enables local regulation of receptor levels by subjugating shedding to the MPs’ spatial distribution or local activation. This attribute seems especially valuable in the case of neural cells, due to the great distances stretched between the soma and the tip of the axon [61] . The in vitro loss of responsiveness of the double-knockout axons at E13.5, as well as their eventual penetration into the spinal cord in vivo , clearly indicates that downregulation of Nrp1 by ADAMs is only part of the equation. Indeed, our biochemical analysis of proprioceptive axons revealed a strong reduction in the total amount of Nrp1.The reduction appears to be MP independent and culminates after desensitization has already been achieved. It seems fair to speculate that the decrease in total Nrp1 reflects the shutting down of cellular mechanisms that replenish receptor levels at the growth cone (for example, transcription, intracellular transport). This may prevent a constant tug of war between Nrp1 cleavage and its membrane trafficking and lock the axons in the unresponsiveness state. Interestingly, such a dual requirement has been demonstrated for the downregulation of the Notch ligand, Delta, in the fly developing wing [62] , [63] . Our experimental data do not reveal whether both ADAM10 and ADAM17 actually cleave Nrp1 under physiological conditions. On the one hand, only simultaneous elimination of the two ADAMs yielded a profound impact on both Nrp1 growth cone levels and axonal repulsion in vitro . On the other hand, the in vivo results suggest that inactivation of ADAM10 alone is sufficient to obtain a robust guidance phenotype. Another indication for the prominent role of ADAM10 may be the hampered ability of the ADAM10 Nrp1 hypercleavable mutant, but not ADAM17 mutant, to desensitize proprioceptive axons to Sema3A. As mentioned earlier, the discrepancies between the in vitro and in vivo data may also reflect the imperfect compatibility between the two. For example, it is possible that additional layers of ADAM regulation, such as expression of tissue inhibitors of metalloproteinase (TIMPs) in the axonal surrounding tissue, are missing in our culture system. Another obvious difference between the two systems relates to the fact that our in vitro experiments are based on axonal re-growth, while the in vivo analysis reflects continuous axonal growth. Nevertheless, despite discrepancies, both in vivo and in vitro results strongly support the involvement of ADAMs in the switch of responsiveness to Sema3A. Finally, the means by which ADAM10 and 17 are themselves regulated in this system remain open for further investigation. Numerous molecular mechanisms have been described for ADAM regulation [13] , [64] . Generally speaking, these can be classified to mechanisms that effect ADAM expression, activity or substrates. An overall increase in ADAM expression, which is ideal for activating multiple targets (for example, during inflammatory response), seems to us less suitable for specifically targeting a single protein. This is underscored by the long list of ADAM10 and 17 substrates that include many neuronally expressed molecules [14] . In agreement, our biochemical analysis suggests that there is no increase in the overall axonal levels of ADAM10 and 17 or in their processing to the mature forms. Thus, we believe that, in the case of Nrp1 shedding, regulation is more likely to rely on the substrate. For example, a change in the composition of proteins surrounding and/or interacting with Nrp1 may cause it to switch conformation that renders it more susceptible to cleavage. The importance of the substrate’s conformation for cleavage was nicely demonstrated for Ephrin-A5, which is cleaved by ADAM10, but only upon forming a complex with its receptor, EphA3 (ref. 23 ). Another plausible mechanism underlying Nrp1 shedding may involve alternative splicing. Interestingly, one of the human Nrp1 splice variants, discovered in endothelial cells and astrocytes, lacks a 17-amino-acid fragment at the juxtamembrane domain [65] . This deletion resides close to the ADAM10 cleavage region that we identified in the rat homologue, and therefore may exhibit altered cleavage properties. If this isoform is indeed expressed in sensory axons, it may also be involved in regulating their differential responses to Sema3A. Thus, further studies are required to define the complement of mechanisms that control the ADAM-mediated cleavage of Nrp1 during development. Animals Pregnant female Wistar rats (8-12 weeks old) were purchased from Harlan (Rehovot, Israel). ADAM10 cKOs, ADAM17 cKOs and ADAM10/17 double cKOs were generated by crossing the previously described ADAM17 lox/lox (ref. 66 ), ADAM10 lox/lox and Nestin-Cre ADAM10 lox/+ (ref. 58 ) lines of mice. Mice were of mix strains and both males and female embryos were used. Mice colonies were bred and maintained at the Department of Veterinary Resources of the Weizmann Institute of Science, Israel, according to recommendations of the Federation of European Laboratory Animal Science Associations. Antibodies For immunofluorescence, the following antibodies were used: human anti-Nrp1 (ref. 67 ) from Genentech (2.2 μg ml −1 ); mouse anti-tubulin βIII (TUJ-1 clone, 1:2,000) from R&D systems; rabbit anti-tubulin βIII (TUJ-1 clone, 1:2,000) from Covance; and mouse anti-Flag M2 from Sigma-Aldrich (1:1,000). Rabbit anti-TAG-1 antibodies (1:1,000) were kindly provided by the lab of Elior Peles (Weizmann Institute of Science). Fluorescent secondary antibodies were purchased from Jackson Immunoresearch. For western blot analysis, the following antibodies were used: biotin-tagged anti-Nrp1 (R&D systems, BAF566, 1 μg ml −1 ) or if specifically indicated in the text—mouse anti-Nrp1 (Abcam, ab16786, 1:100); Rabbit anti-ADAM10 (Abcam, ab1997, 2 μg ml −1 ); Rabbit anti-ADAM17 (Millipore, AB19027, 1:1,000); mouse anti-Flag M2 from Sigma-Aldrich (1:1,000); and mouse anti-Myc (D9 hybridoma, 1:1,000) from the Weizmann Institute antibodies unit. HRP-conjugated secondary antibodies were purchased from Jackson Immunoresearch. For immunohistochemical staining goat anti-TrkC (AF1404, R&D systems, 2 μg ml −1 ) and donkey anti-goat Cy3 (Jackson Immunoresearch, 1:300) were used. Plasmids, cloning and mutagenesis Mouse ADAM10 and rat ADAM 8,9,15 and 17 were cloned into psecTAG-B vector (Invitrogen) in frame with a Myc tag at their C-terminal ends. Nrp1 insertion mutants were generated by adding the Myc epitope at the indicated sites using Stratagene’s QuikCange technique. Nrp1 deletion mutants were generated using ‘back-to-back’ primers, designed to amplify the entire plasmid, excluding the desired omission [68] . In the neuronal overexpression experiments pCAGGS/ES vectors (harbouring beta actin promoter), encoding Nrp1 variants (wild type, ADAM10 hyper-cleavable, ADAM17 hyper-cleavable), as well as L1-CAM, were used. For the co-immunoprecipitation experiments C-terminally HA-tagged Nrp1 and 2 and C-terminally Myc-tagged Plexin-A1 and N-terminally Myc-tagged Plexin-A4 were used. Immunostaining For rat immunostaining experiments, DRGs from E13, E14 and E15 embryos were dissected (all at the same day). For the mouse immunostaining experiments, DRGs were dissected from E11.5 and/or E12.5 wild type and mutant embryos (only littermates were compared). Overall, 3–4 separate experiments were performed for rat and 3–7 for mouse. Explants were cultured on 13 mm coverslips (eight DRGs per coverslip) that were pre-covered with poly D -lysine (10 μg ml −1 , Sigma-Aldrich, 2 h at room temperature) and laminin (10 μg ml −1 , Sigma-Aldrich, 2 h at 37 °C). Culture media consisted of Neurobasal-A medium (Gibco), 1 × B-27 (Gibco), 2 mM glutamine (Biological Industries, Israel), penicillin-streptomycin (Biological Industries, Israel) and either 50 ng ml −1 NT3 (PeproTech) or 12.5 ng ml −1 NGF (Alomone). The general metalloprotease inhibitor TAPI-1 (20 μM, Merck-Millipore) or equivalent volume of DMSO (carrier) was also added to the media, as indicated. After 18 h incubation the cultures were fixed with 4% paraformaldehyde, 15% sucrose in PBS solution and stained with anti-Nrp1 and anti-TAG-1 antibodies. Immunostained DRGs were visualized by the Nikon Eclipse 90i microscope and quantified using the NIS-elements AR 3.2 imaging software. Average fluorescence of each growth cone was determined using the NIS-elements rectangle tool (for each growth cone the largest inscribed rectangle was selected). All growth cones with average fluorescent values lower than 10 times the background level were discarded. In the rat experiments, 1,200–4,500 growth cones were measured for each reported condition. In each experiment, the average fluorescence of all E13 growth cones, cultured without TAPI-1, was calculated and arbitrarily set to 1. All other measurements in the same experiment were normalized relative to it. In the mouse experiments 1,200–5,500 growth cones were measured for each condition. Average fluorescence of E11.5 wild-type growth cones, cultured without TAPI-1, was arbitrarily set to 1, and all other measurements were normalized relative to it. To validate the quantification method, selected sets of pictures were re-quantified. These repeated measurements yielded less than 2% difference relative to the original measurements. Analysis of supernatants HEK293T cells were divided into six-well plates and cultured in DMEM medium (Gibco), added by 2 mM glutamine and penicillin-streptomycin antibiotics. The cells were transiently transfected with plasmids encoding wild type or mutant rat Nrp1 together or without different members of the ADAM family, using Jet-PEI transfection reagent (Polyplus Transfection). After 24 h incubation, the medium was replaced by serum-free F12/DMEM medium (Biological Industries, Israel), supplemented with glutamine and penicillin-streptomycin. When necessary, the serum-free medium was also supplemented with pharmacological inhibitors or equivalent volume of DMSO for the controls. After another 24 h, Supernatants were collected and briefly centrifuged to dispose of residual cell debris. Then, supernatants were resolved on 8% SDS-PAGE (Biological Industries, Israel) gel and analysed by western blot. In parallel, cells extracts were prepared by adding 0.3 ml 1 × RIPA buffer, supplemented with 1 mM PMSF (Sigma Aldrich) and 1 × Complete protease inhibitor cocktail (Roche) to each well after conditioned medium collection. After 10 min incubation on ice, HEK293T cells were scrapped and transferred into eppendorf tubes for another 30 min incubation, accompanied by occasional vortex. Finally, cell debris was removed by centrifugation (20 min, 14,000 r.p.m., 4 °C), and supernatants collected and analysed by western blot. Collagen repulsion assay Collagen repulsion assays were performed as previously described [69] . In brief, DRGs were dissected at the indicated embryonic day from either rat or mouse embryos. The DRGs were placed in droplets of 2 mg ml −1 collagen (Roche), next to Sema3A-secreting aggregates, and cultured in F12/Opti-MEM medium, comprised of F12 (Biological Industries, Israel)/Opti-MEM (Gibco) (1:2 v/v ratio), 40 mM dextrose (Sigma-Aldrich), 2 mM glutamine, penicillin-streptomycin and supplemented with 50 ng ml −1 NT3 or 12.5 ng ml −1 NGF. The aggregates for the assay were produced by mixing COS-1 cells, previously transfected with Sema3A encoding plasmids, with concentrated collagen (10 mg ml −1 , Becton Dickinson) (1:1 v/v ratio), and incubating at 37 °C/5% CO 2 for 30 min. After 36–48 h (for rat DRGs) or 48–60 h (for mouse DRGs) the co-cultures were fixed with 4% formaldehyde, stained using mouse anti-tubulin βIII antibodies and visualized by the Leica MZ16F microscope. Proximal/distal (P/D) ratio quantifications were performed by a Matlab program, designed according to the following guidelines: for each DRG, axonal growth was examined within two quadrants, ranging between ±45° around the horizontal axis on both proximal and distal sides of the explant (see Fig. 1e ). Each quadrant was divided into 630 equal angular segments (1/7° each). Longest axon within each segment was computationally identified, and the distance from its tip to the surface of the DRG was measured. This measurement was defined as the axonal length of that particular segment. Total axon length, for either proximal or distal sides of the explant, was determined by summing up all axonal lengths within the relevant quadrant. Finally, the ratio between proximal and distal total axon lengths was calculated for each DRG and used as an indicator for sensitivity to Sema3A. Preparation of axonal extracts Cell culture inserts (fit for six-well plate, PET membrane, 1 μm pore size, Becton Dickinson) were coated on both sides with poly D -lysine (10 μg ml −1 , Sigma-Aldrich, 2 h at room temperature) and laminin (10 μg ml −1 , Sigma-Aldrich, 2 h at 37 °C). Each insert was placed inside a well, containing 2 ml of F12/Opti-MEM medium with 50 ng ml −1 NT3 or 12.5 ng ml −1 NGF. The inner side of the insert was filled with 1 ml of the same medium. Whole DRGs, extracted from rat embryos at the indicated developmental stage, were placed inside the inserts (50–100 DRGs per insert) and cultured for ~36 h, allowing the axons, but not cell bodies, to pass through the pores and grow on the bottom surface of the insert. Finally, each side of the insert membrane was separately lysed and scraped in 100 μl (axons) or 200 μl (cell bodies) of 1 × RIPA buffer (supplemented with 1 mM PMSF and 1 × Complete protease inhibitor cocktail). The lysate-containing buffer was transferred into eppendorf tubes for 30 min (accompanied by occasional vortexing), and cell debris was removed by centrifugation (20 min, 14,000 r.p.m., 4 °C). Electroporation and neuronal aggregation DRGs were dissected from E14 rat embryos and pelleted in Hank’s balanced salt solution (Biological Industries, Israel). The cells were trypsinized (0.25% Trypsin-EDTA solution B, Biological Industries, Israel), neutralized by L-15 medium (Sigma-Aldrich) supplemented with 5% fetal bovine serum (BI), and finally triturated by repeated pipettation. Electroporation was performed using the Amaxa Nucleofector 96-well shuttle according to the manufacturer’s instructions. In brief, DRG dissociated cells were pelleted and re-suspended in supplemented P3 primary cell solution (250,000 cells/20 μl solution) of the Amaxa electroporation kit (cat# V4SP-3096, Lonza). After addition of the desired plasmid (1 μg plasmid/250,000 cells), the cell solution was transferred to the Nucleofector 96-well plate (20 μl solution per well) and electroporated using the 96-CA-138 nucleofection programme. Immediately, Neurobasal-A medium—supplemented with 1 × B-27, 2 mM glutamine, penicillin-streptomycin, 10% fetal bovine serum and 50 ng ml −1 NT3, and pre-heated to 37 °C—was added to each well to allow recovery of the electroporated cells. For the preparation of neuronal aggregates 500,000–750,000 electroporated DRG cells were pelleted and re-suspended in 10 μl of Neurobasal-A medium (supplemented with foetal bovine serum and NT3). The re-suspended cells were injected into a ‘hanging drop’ of the same medium (20 μl in volume) and incubated at 37 °C overnight. The following day, the aggregated neuronal mass was dissected into smaller aggregates that were used in collagen assays as described above for DRGs. Immunohistochemistry Spinal cords of E12.5-E14.5 wild type and ADAM-knockout mouse embryos were dissected, washed in PBS and fixated in 4% formaldehyde (2–3 h, room temperature). After fixation, the spinal cords were washed again in PBS and transferred to 30% sucrose solution (in PBS) for overnight incubation (4 °C). Next, the explants were incubated for 30 min (room temperature) in O.C.T (Tissue-Tek, Sakura), transferred to embedding molds containing O.C.T, and quickly frozen in ethanol bath containing dry ice. Molds were kept at −80 °C until sectioning. Transverse slices (25 μm width) from spinal cord cervical regions were prepared using cryostat microtome and mounted on slides. Slides were left at room temperature for 1 h, washed three times in PBS and blocked with 1% BSA, 0.2% Triton in PBS (2 h, wet chamber at room temperature). Next, slides were incubated for 2 h with an anti-TrkC antibody (see above), washed three times in blocking solution and incubated for another 2 h in the Cy3-conjugated secondary antibody. Finally, slides were washed three times in blocking solution and once more in PBS and covered with cover glass. Seam3A binding assay COS7 cells were transfected with wild-type Nrp1 and hyper-cleavable mutant constructs and cultured for 24 h at 37 °C/5% CO 2 . Transfected and parental cells were washed with HBSBA buffer (20 mM HEPES pH=7, 5 mM CaCl 2 , 1 mM MgCl 2 , 0.2% BSA and 0.1% NaN 3 ) and incubated at room temperature with increasing concentrations of Sema3A-AP-containing culture medium and 2 μg ml −1 Heparin (Sigma) for 90 min. After the removal of unbound ligands, cells were lysed with lysis buffer (10 mM Tris pH=9.5, 1% Triton and Protease Inhibitors) and the AP activity was measured in AP buffer (1 M Diethanolamine pH=9.8, 0.5 mM MgCl 2 and 50 mg p -nitrophenylphosphate) at 405 nM. Co-immunoprecipitation Myc-tagged Plexin-A1 or Plexin-A4, or HA-tagged Nrp1 or Nrp2 were co-transfected into HEK293T cells (cultured in six-well plates) with Flag-tagged Nrp1 (wild-type or hypercleavable mutant), or empty vector, as indicated. After 24–48 h incubation, 500 μl of solubilization buffer (50 mM HEPES pH 7.5, 150 mM NaCl, 10% glycerol, 1% Triton, 5 mM EGTA, 1 mM PMSF and 1 × Complete protease inhibitor cocktail) was added to each well. After 10 min incubation on ice, cells were scrapped and collected into eppendorf tubes. Extracts were left on ice for 2 h (with occasional pipetting), and eventually cell debris was removed by 20 min centrifugation (14,000 r.p.m., 4 °C). Then, each tube was incubated overnight (on tube rotator, 10 r.p.m., 4 °C) with 2 μl anti-Flag antibody, The following day, each tube was further supplemented with ~30 μl of protein A/G-Agarose beads (sc-2003, Santa Cruz), pre-washed with ice-cold PBS and left to rotate for 1 h at 4 °C. Then, the beads were pelleted (1 min, 10,000 g , 4 °C) and washed twice in 1 ml cold PBS. Following the final centrifugation, supernatants were discarded and pellets were resuspended in 1 × sample buffer, boiled for 5 min and loaded onto 8% SDS-PAGE gel. Finally, the gel was immunoblotted with antibodies against the Myc or HA epitopes. Whole-mount neurofilament staining E12.5 wild type and ADAM10/17 double-knockout embryos were collected in PBS, and fixated in 4% formaldehyde (2–3 h, room temperature). After three washes (10 min each) in PBS with 0.2% Triton, embryos were dehydrated in increasing concentrations of methanol in PBS (10, 30, 50 and 80%, 1 h incubation for each concentration). After dehydration, embryos were bleached in 80% methanol/ 6% H 2 O 2 (Merck) (overnight, 4 °C), washed three times in 80% methanol (in PBS) and rehydrated in 50, 30 and 10% methanol (1 h each wash). After another three washes of 30 min in PBS with 0.2% Triton, embryos were left in blocking solution (2% milk powder, 0.2% Triton in PBS) overnight (4 °C). Then, they were further incubated with the mouse anti-neurofilament antibody (2H3, DSHB, 1:200) for 3 days at 4 °C. After six washes in blocking solution (1 h each), embryos were transferred to secondary antibody solution (HRP-coupled goat anti mouse 1:200 in blocking solution supplemented with 2% heat-inactivated goat serum) for overnight incubation. Before developing, embryos were washed four times in blocking solution with 2% goat serum, and twice in PBS with 0.2% triton (1 h each wash), and incubated for 30 min in 0.1 M Tris pH7.5 solution supplemented with 3,3′-Diaminobenzidine tetrahydrochloride (DAB, Sigma-Aldrich, 1 tablet per 15 ml) that was pre-filtered using a 0.45-μm syringe filter. Embryos were developed in 0.1 M Tris pH 7.5/DAB solution supplemented with 0.5% NiCl 2 (Sigma Aldrich) and 0.03% H 2 0 2 , and stopped by two rinses in PBS, 10 min incubation in 4% formaldehyde and finally three rinses in PBS. How to cite this article: Romi, E. et al. ADAM metalloproteases promote a developmental switch in responsiveness to the axonal repellant Sema3A. Nat. Commun. 5:4058 doi: 10.1038/ncomms5058 (2014).